Volcano seismicity and ground deformation unveil the gravity-driven magma discharge dynamics of a volcanic eruption Effusive eruptions are explained as the mechanism by which volcanoes restore the equilibrium perturbed by magma rising in a chamber deep in the crust. Seismic, ground deformation and topographic measurements are compared with effusion rate during the 2007 Stromboli eruption, drawing an eruptive scenario that shifts our attention from the interior of the crust to the surface. The eruption is modelled as a gravity-driven drainage of magma stored in the volcanic edifice with a minor contribution of magma supplied at a steady rate from a deep reservoir. Here we show that the discharge rate can be predicted by the contraction of the volcano edifice and that the very-long-period seismicity migrates downwards, tracking the residual volume of magma in the shallow reservoir. Gravity-driven magma discharge dynamics explain the initially high discharge rates observed during eruptive crises and greatly influence our ability to predict the evolution of effusive eruptions. First defined as the instantaneous flow output of a vent [1] , the lava effusion rate is now regarded as a vital parameter for interpreting eruptive dynamics and for hazard management during volcanic crises. Most basaltic eruptions are characterized by exponential decays in the effusion rate, which are explained by the tapping of a pressurized reservoir [2] , [3] . The origin of the rapid lava discharge rate in the initial phase of the eruption, as well as the overpressure of the magmatic reservoir, is unclear, and this has a strong impact on our ability to reliably assess the associated risks. Similar to eruptions at other basaltic volcanoes, the effusion rate of the February 2007 eruption of the Stromboli volcano (Aeolian Archipelago, Southern Italy) exhibits a rapid exponential decay characterized by an initial discharge rate of 23 m 3 s −1 that rapidly dropped to ∼ 3 m 3 s −1 within a few days [4] , [5] , [6] , [7] . Although the measurement of effusion rates is a challenge at the best of times, in the case of the 2007 Stromboli eruption, the rate was measured using the thermal data from two different satellites (Advanced Very High Resolution Radiometer (AVHRR) and Moderate Resolution Imaging Spectroradiometer (MODIS)), which were compared with ground-based thermal [8] and topographic laser scanner measurements [6] . One week after the eruption onset (7 March) the crater terrace collapsed, forming a ∼ 300-m-long by ∼ 140-m-wide caldera [5] , [6] with major consequences for the stability of this potentially tsunamogenic structure [9] . High magma effusion rates can in fact trigger instability in the steep slope flanks of volcanic edifices [10] , [11] . On 15 March, as a possible final consequence of the effusive dynamics, a violent ‘paroxysmal’ explosion several orders of magnitude larger than normal Strombolian activity occurred and metre-sized bombs hit the two nearby villages ∼ 2 km from the craters [12] . The eruption finally ceased on 2 April 2007 after erupting 8.2±1.5 × 10 6 m 3 of dense rock equivalent (DRE) lava in 34 days [6] , [8] . This eruption offered a unique opportunity to analyse the evolution of the effusive regime and to understand the link between geophysical parameters and the effusive dynamics. We show that the effusion rate can be measured by ground deformation, which coincides with the contraction of the volcano, and that the magma level within the conduit can be successfully tracked by the lowering of the very-long-period (VLP) seismicity during the effusive event, presenting a useful method for monitoring the real-time evolution of effusive volcanic eruptions. Migration of the VLP seismic source This eruption was monitored by a large number of geophysical and geochemical sensors, including a broad-band seismic station and two tiltmeters (stations STR, LSC and OHO, respectively, in Fig. 1a ). Volcanic activity was also recorded with a thermal camera (station ROC in Fig. 1a ) located on the northeast flank of the volcano at an elevation of 650 m a.s.l. (above sea level) and at a distance of ∼ 500 m from the active vents. 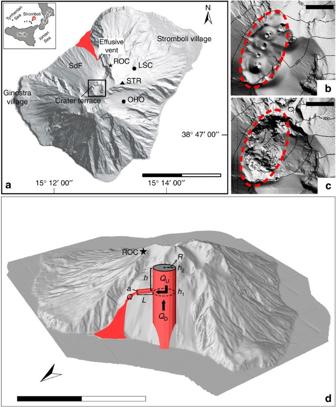Figure 1: (a) Shaded relief map of Stromboli with the main lava flow during the 2007 eruption and position of the lateral effusive vent at 400 m elevation in the Sciara del Fuoco (SdF). Scale bar, 2 km. Location of the geophysical network operating during the 2007 eruption: the star (ROC) indicates the position of the thermal camera (uncooled microbolometer FLIR-A20), the triangle (STR) represents the position of the broad-band seismic station (CMG-40T, 800 V m−1s−1, eigenperiod 30 s), and the circles (LSC and OHO) mark the two tiltmeters (Pinnacle 5000T sampled at 1 Hz and with a sensitivity of 1 nrad). The black square delimits the area represented inbandc. (b) Close-up of the crater area before the 7–9 March 2007 crater terrace collapse. (c) Crater area after the collapse (red dashed line). Scale bars, 100 m (b,c). (d) The volcano seen from the north, with a sketch of the shallow reservoir with the parameters used to calculate the discharge model. Scale bar, 2 km.QUrepresents the supply rate from the reservoir above the lateral vent,QD(0.7 m3s−1) is the steady magma supply rate from depth,Qis the effusive rate from the lateral vent,a(1.5 m) is the radius of the effusive channel,L(98–154 m) is the length of the channel,his the magma level above the effusive vent (286–363 m) andR(95±5 m) is the radius of the reservoir within the considered vesicularity range of 0.14 and 0.45.bandcare redrawn after6. Figure 1: ( a ) Shaded relief map of Stromboli with the main lava flow during the 2007 eruption and position of the lateral effusive vent at 400 m elevation in the Sciara del Fuoco (SdF). Scale bar, 2 km. Location of the geophysical network operating during the 2007 eruption: the star (ROC) indicates the position of the thermal camera (uncooled microbolometer FLIR-A20), the triangle (STR) represents the position of the broad-band seismic station (CMG-40T, 800 V m −1 s −1 , eigenperiod 30 s), and the circles (LSC and OHO) mark the two tiltmeters (Pinnacle 5000T sampled at 1 Hz and with a sensitivity of 1 nrad). The black square delimits the area represented in b and c . ( b ) Close-up of the crater area before the 7–9 March 2007 crater terrace collapse. ( c ) Crater area after the collapse (red dashed line). Scale bars, 100 m ( b , c ). ( d ) The volcano seen from the north, with a sketch of the shallow reservoir with the parameters used to calculate the discharge model. Scale bar, 2 km. Q U represents the supply rate from the reservoir above the lateral vent, Q D (0.7 m 3 s −1 ) is the steady magma supply rate from depth, Q is the effusive rate from the lateral vent, a (1.5 m) is the radius of the effusive channel, L (98–154 m) is the length of the channel, h is the magma level above the effusive vent (286–363 m) and R (95±5 m) is the radius of the reservoir within the considered vesicularity range of 0.14 and 0.45. b and c are redrawn after [6] . Full size image The transition from the persistent Strombolian explosive activity to the effusive regime began on 27 February 2007 (ref. 13 ) when a well-supplied lava effusion began to flow from a lateral vent at 400 m a.s.l. within the Sciara del Fuoco slope and explosive activity at the summit craters suddenly ceased ( Fig. 1 ). However, the VLP seismicity commonly associated with the explosive activity was uninterrupted [14] . Despite the transition to effusive activity and the absence of Strombolian explosions, the VLP volcanic seismicity remained intense [13] , [14] . The location of VLP seismicity in Stromboli is in general considered to be stable at ∼ 500 m a.s.l. [15] , which corresponds to a depth of 220–300 m below the active craters. This depth represents the position of the centroid of the seismic moment inversion [15] and is interpreted as a change in conduit geometry (a dyke merging into a pipe or a change in the dyke slope), which is responsible for the sudden expansion of the gas slug [15] , [16] that eventually explodes upon reaching the magma surface. Here, we present evidence that forces us to change this scenario of stability and that opens questions on the origins of this seismic signal. The relative changes of source location can be tracked by calculating the orientation of the ground displacement particle motion vector that represents the propagation path of the longitudinal P-wave component of the VLP events [17] . Due to the uncertainty in seismic velocity structure and in the curvature of the P-wave path, the inclination in the displacement vector cannot directly deduce absolute changes in the VLP source position, but can be considered to be an efficient tracer of the relative movement of the source. The displacement vectors of ∼ 300,000 seismic VLPs recorded at STR ( Fig. 1a ) between January 2006 and January 2008 ( Fig. 2a ) exhibit a stable inclination of within ∼ −4° below the station until the beginning of February 2007. At the onset of the eruption, the inclination of the vector changes and progressively moves downwards, reaching ∼ −13° at the end of the eruption on 2 April ( Fig. 2a ). At this time, the inclination of the ground displacement vector begins to move upward again, reaching a stable position of ∼ −9° on 1 May ( Fig. 2a ). 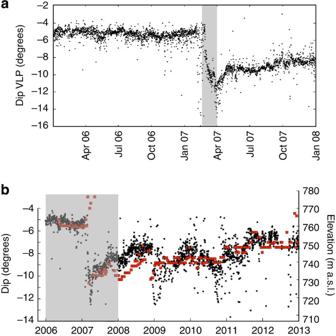Figure 2: (a) Dip of the ground displacement vector calculated for 280,548 VLP seismic events recorded at STR (seeFig. 1a) between January 2006 and January 2008. Dip is measured from the horizontal plane defined by the station elevation and remained almost stable at approximately −5° until the onset of the eruption. On 27 February 2007, the VLP source shifts progressively deeper to −13° until 2 April 2007, when the VLP source shifts back towards the surface. Position becomes stable at −9° on 1 May 2007, but the pre-eruptive conditions have not yet been reached. The grey area represents the duration of the 2007 eruptive phase. (b) Seven years of displacement vector inclinations (black dots) are compared with the elevation of the crater rim (red squares), as measured by the thermal camera at ROC. The correlation suggests that the position of the seismic source is constrained by the topography and reflects changes in the magma level in the shallow conduits. In 2013, 6 years after the eruption, the 2.1 × 106-m3caldera (Fig. 1c) has not been totally filled. The grey area represents the time window shown ina. Figure 2: ( a ) Dip of the ground displacement vector calculated for 280,548 VLP seismic events recorded at STR (see Fig. 1a ) between January 2006 and January 2008. Dip is measured from the horizontal plane defined by the station elevation and remained almost stable at approximately −5° until the onset of the eruption. On 27 February 2007, the VLP source shifts progressively deeper to −13° until 2 April 2007, when the VLP source shifts back towards the surface. Position becomes stable at −9° on 1 May 2007, but the pre-eruptive conditions have not yet been reached. The grey area represents the duration of the 2007 eruptive phase. ( b ) Seven years of displacement vector inclinations (black dots) are compared with the elevation of the crater rim (red squares), as measured by the thermal camera at ROC. The correlation suggests that the position of the seismic source is constrained by the topography and reflects changes in the magma level in the shallow conduits. In 2013, 6 years after the eruption, the 2.1 × 10 6 -m 3 caldera ( Fig. 1c ) has not been totally filled. The grey area represents the time window shown in a . Full size image This change in VLP source position is also confirmed by the analysis of 11 broad-band seismic stations [14] and was also observed during the 2003 eruption [17] . The drift of the VLP seismicity appears to follow the drainage of the magma during the effusive eruption. These observations are difficult to reconcile with the previous image of a stable VLP source in the central conduit [15] and cannot be explained with effusive dynamics solely sustained by the magma supply rate from depth. Volume of lava discharged and VLP source migration The effusion rate Q ( t ) can be converted into the magma volume resident in the reservoir, where V 0 =8.2±1.5 × 10 6 m 3 is the total erupted volume of DRE magma ( Supplementary Table 1 ). The residual magma volume V R represents the way the reservoir progressively empties during the eruption. The measured volume of magma V R ( t ) yet to be discharged correlates well ( R 2 =0.93) with the migration trend of the VLP displacement vector ( Fig. 3 ). This linear correlation ( Fig. 3 inset) provides remarkable evidence for a link between the volume of magma discharged and the vertical position of the VLP seismicity, indicating that the effusive volume decreases linearly with depth. This provides a strong constraint on the geometry and position of the reservoir. The reservoir can thus be represented by a shallow cylindrical plumbing system immediately above the effusive vent, with the same area as the crater terrace, A 0 ∼ 3.0±0.2 × 10 4 m 2 (equivalent to an ellipse ∼ 300 m long by ∼ 140 m wide, Fig. 1c ). 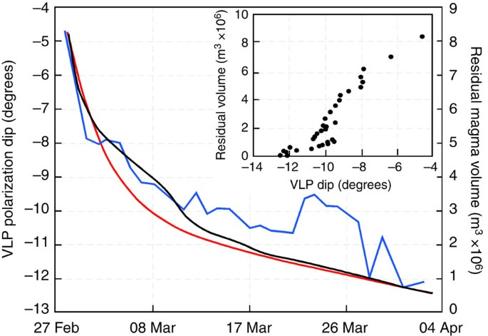Figure 3: The migration of the VLP inclination vector (blue line) measured during the eruption (grey band inFig. 2a) is compared with the residual magma volume in the upper cylindrical reservoir (black line) by assuming the measured effusion rate and with the discharge model (equation (1)) controlled by the drainage of magma stored above the vent (red line). The inset shows the remarkably good (R2=0.93) correlation between the level of magmah(t) in the reservoir and the seismic source dip. In this case, the residual volume, V R ( t ), can be converted to changes in the magma level in the reservoir: Figure 3: The migration of the VLP inclination vector (blue line) measured during the eruption (grey band in Fig. 2a ) is compared with the residual magma volume in the upper cylindrical reservoir (black line) by assuming the measured effusion rate and with the discharge model (equation (1)) controlled by the drainage of magma stored above the vent (red line). The inset shows the remarkably good ( R 2 =0.93) correlation between the level of magma h ( t ) in the reservoir and the seismic source dip. Full size image where is the magma vesicularity ranging between 0.14 and 0.45 (ref. 18 ). With this geometry, we calculate that the change in the residual magma volume reflects a total lowering of the magma level in the conduit of 286 and 363 m below the surface, within the considered magma vesicularity range. Both cases indicate that the magma level before the eruption was very shallow, between 686 and 763 m a.s.l. The VLP source location thus tracks the position of the magma level in the conduit during the effusive eruption, which has significant consequences for our understanding of the VLP source mechanisms and for volcano monitoring in general. When the eruption ceased on 2 April, the position of the VLP seismicity moved upwards, reaching a stable dip of −9°. This inclination is ∼ 5° deeper than before the eruption ( Fig. 2a ), suggesting that the magma level only partially recovered its initial position. This observation is consistent with the lower elevation of the craters after the eruption ( Fig. 1b,c ), due to the ∼ 65 m of subsidence in the terrace floor [6] . The topographic elevation of the crater floor limits the position of the magma level and appears to limit the level and the depth of the VLP seismicity within the conduit, as we now discuss. Tracking crater growth and VLP seismicity Using thermal image analysis, we tracked the evolution of the crater terrace from January 2006 until January 2013. The deposition of hot scoria ejected by the persistent explosive activity falling on the crater rim provided a strong thermal contrast between the ground and the cold background sky, allowing the tracking of the crater terrace’s elevation changes through time. The thermal image analysis shows that the position of the craters remained at a stable elevation of ∼ 760 m a.s.l. until the onset of the eruption ( Fig. 2b ). During the 7–9 March collapse, the crater terrace dropped far below the field of view of the thermal camera. After 2 April 2007, at the eruption’s end, the thermal camera again detected the growth of the crater terrace as a consequence of the resumed explosive activity at the vent. Remarkably, changes in the topographic elevation of the craters are associated with the variations in the VLP seismicity position ( Fig. 2b ), confirming the link between the VLP seismicity and the magma level within the conduit. In 2013, 6 years after the eruption, the pre-eruptive elevation of the crater terrace has still not entirely recovered. The elevation of the explosive vents is at ∼ 750 m a.s.l., ∼ 10 m lower than the level prior to 2007, and the VLP seismicity has not totally returned to the ∼ 5° pre-eruptive inclination ( Fig. 2b ). During these 6 years, the large ∼ 2.1 × 10 6 -m 3 caldera-like structure [6] has been partially filled with scoria and bombs by explosive activity, with a mean magma output rate of ∼ 0.01 m 3 s −1 . This is consistent with the characteristic rate of Strombolian activity characterized by 10 explosions per hour, each ∼ 3.6 m 3 in size [13] , [19] . Modelling the gravity-driven lava discharge rate The effusion rate, Q U ( t ) =πa 2 u ( t ), decays in time depending on the exit velocity, u ( t ), of the lava flow from the vent with radius a (1.5 m in our case [20] ). Modelling the effusion rate means modelling changes in the exit velocity with time. The exponential decay of the effusion rate can be modelled by assuming that gravity is draining magma out of the reservoir through a dyke-like channel of length L with exit velocity controlled by Poiseuille flow in the channel [2] : where η is the magma viscosity of 10 4 Pas [21] . Because the magma was near the surface before the eruption [4] , [9] , we use the relationship ΔP ( t )= P h ( t ) −P atm to calculate the pressure difference between the magmastatic pressure of the reservoir, P h ( t ) =ρgh ( t )( 1−φ ), and the atmospheric pressure at the vent, P atm =10 5 Pa, where h ( t ) is the gradual reduction of the magma level above the effusive vent (equation (1)) and ρ =2,950 kg m −3 is the DRE magma density [22] ( Supplementary Table 1 ). The modelled extrusion rate, Q U ( t ), exhibits the best fit with the observed extrusion rate ( Fig. 4 ) and with the volumetric discharge associated with the migration of the VLP seismicity ( Fig. 3 ) for a channel length L , ranging between 98 and 154 m in the assumed vesicularity range ( Fig. 1d ). 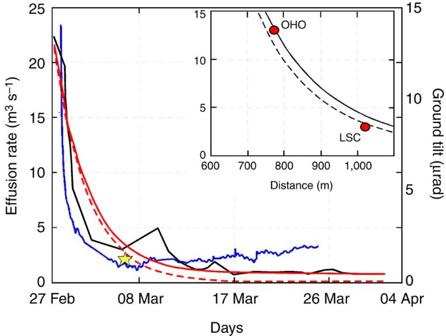Figure 4: Comparison between the ground tilt at the OHO station (blue), the observed effusion rate (black) and modelled discharge (red). The model (equation (1)) assumes a steady deep magma supply rate (QD) of 0.7 m3s−1and a shallow plumbing system represented by a cylindrical reservoir immediately above the effusive vent, with the same area as the crater terrace,A0=3.0±0.2 × 104m2. When no deep magma is supplied (QD=0; red dashed line), the discharge rate of the shallow reservoir goes to zero after 18 days following the eruption onset. A value ofQD=0.7 m3s−1is consistent with the SO2flux measured during the eruption16. The yellow star indicates the change in the effusion rate measured during the eruption, which coincides with the maximum ground deflation (13 μrad) detected by a tiltmeter and with the collapse of the crater terrace. Inset: the ground tilt, modelled (equation (4)) as the magmastatic pressure drop of 6.7 and 4.3 MPa and assuming a vesicularity range of 0.14 (dashed line) and 0.45 (bold line), respectively, gives the best fit with the maximum ground deflation observed at both OHO and LSC stations (red dots). This corresponds to the lowering of the magmatic column by 330±20 m. Figure 4: Comparison between the ground tilt at the OHO station (blue), the observed effusion rate (black) and modelled discharge (red). The model (equation (1)) assumes a steady deep magma supply rate ( Q D ) of 0.7 m 3 s −1 and a shallow plumbing system represented by a cylindrical reservoir immediately above the effusive vent, with the same area as the crater terrace, A 0 =3.0±0.2 × 10 4 m 2 . When no deep magma is supplied ( Q D =0; red dashed line), the discharge rate of the shallow reservoir goes to zero after 18 days following the eruption onset. A value of Q D =0.7 m 3 s −1 is consistent with the SO 2 flux measured during the eruption [16] . The yellow star indicates the change in the effusion rate measured during the eruption, which coincides with the maximum ground deflation (13 μrad) detected by a tiltmeter and with the collapse of the crater terrace. Inset: the ground tilt, modelled (equation (4)) as the magmastatic pressure drop of 6.7 and 4.3 MPa and assuming a vesicularity range of 0.14 (dashed line) and 0.45 (bold line), respectively, gives the best fit with the maximum ground deflation observed at both OHO and LSC stations (red dots). This corresponds to the lowering of the magmatic column by 330±20 m. Full size image However, in both cases, the predicted effusion rate quickly decays to zero ( Fig. 4 , dashed red line) and the model is not able to fully reproduce a long-lasting effusive eruption. The model indicates that magma supplied from depth should be considered a damping factor in the drainage dynamics of the shallow reservoir and that this supply provides an important contribution to sustaining the eruption. The extrusion rate Q ( t ) =Q U ( t ) +Q D can be considered the result of the magma drainage Q U ( t ) from the reservoir above the effusive vent and the magma supply rate Q D from depth. The total extrusion rate is then successfully modelled ( Fig. 4 ) only when a steady contribution of Q D =0.7 m 3 s −1 of magma supplied from depth is considered, in addition to the gravity-driven (equation (1)) discharge dynamics of the shallow reservoir Q U ( t ) below the crater terrace. This is in agreement with gas flux measurements [23] , [24] . The SO 2 flux, in fact, increased from an average of 220 t per day before the eruption to 610 t per day during the eruption [23] , a sign that magma was supplied from depth at a rate ∼ 2.7 times higher during the eruption than before. Considering the characteristic mean pre-eruptive magma supply rate of 0.28 m 3 s −1 (ref. 23 ), the increase of SO 2 flux is consistent with a deep magma supply rate of ∼ 0.75 m 3 s −1 during the eruption, which is similar to the rate predicted by the modelling. Modelling ground deformation by effusion rate The rapid decay of the extrusion rate correlates well with the ground deformation ( Fig. 4 ) recorded by the tiltmeters located at distances of 765 m (OHO at an elevation 570 m a.s.l.) and 1,015 m (LSC at an elevation of 520 m a.s.l.) from the active vents ( Fig. 1a,d ). The largest ground deformation, −13 μrad at OHO and −2.8 μrad at LSC, is reached between 7 and 9 March ( Fig. 4 ), and it coincides with the collapse of the floor of the crater terrace. Because the ground deformation is driven by the effusive drainage of magma, as a first approximation, we model the ground tilt ( τ ) as the result of the normal stress acting on the wall of the cylindrical open conduit [25] , [26] of radius R =95±5 m (which is the equivalent of the surface area of the crater terrace): where μ is the rigidity, with a value of 1.3 × 10 9 Pa [27] and G is a parameter, which depends on the relative position of the conduit with respect to the stations ( Supplementary Note 1 ). This source contracts following the pressure difference Δ P related to the effusion rate Q ( t ) modelled as magmastatically driven Poiseuille flow [28] (equation (1)). The expected ground tilt induced by the measured effusion rate ( Fig. 4 ) is then calculated as follows: where ΔQ ( t ) =Q 0 −Q ( t ) is the change in effusion rate with time ( Q 0 =23 m 3 s −1 ). Although the trend of the modelled tilt τ ( t ) obviously resembles the effusion rate Q ( t ), the best fit with the absolute measured ground tilt at the two stations [26] (OHO and LSC) is reached for a magmastatic decompression of 6.7 and 4.3 MPa relative to a vesicularity of 0.14 and 0.45 (ref. 18 ), respectively ( Fig. 4 inset). We do not consider in this analytic solution the steep volcano topography; however, the ground deformation, in agreement with the gravity-driven magma discharge model, is reasonably explained by the 330±20-m lowering of the magma in the shallow reservoir located above the effusive vent. This hypothesis provides a useful way to calculate the effusion rate during an eruption in real time. The largest contraction of the source was reached between 7 and 9 March, when ∼ 66% of the total volume stored in the shallow portion of the conduit had already been erupted, and this contraction coincided with the largest modelled magma level drop and with the collapse of the crater terrace. During normal explosive activity, magma flows within the conduits of the Stromboli volcano at a rate of ∼ 0.3 m 3 s −1 (ref. 29 ), but the explosive mechanisms release only a small fraction of the long-term magma supply rate from depth ( ∼ 0.01 m 3 s −1 ). The explosive activity does not evacuate all the magma supplied, which is thus slowly stored at shallow depth and possibly recycled within the plumbing system in which it evolves and crystallizes [21] . This mechanism explains why there was no clear evidence of ground inflation in the days, months and years preceding the eruption [30] , [31] . The high gas flux measured during lava effusion [23] , [24] indicates the increased contribution of a gas-rich, deep-seated magma, and is suggested to be responsible for the increase in magma vesicularity within the shallow reservoir [23] . The discharge of magma during the effusive eruption probably hampered the recycling of the degassed magma, leading to a decrease in the bulk magma density of the shallow plumbing system [23] . This hypothesis explains the contraction of the intermediate depth (2–3 km) magma reservoir observed by ground deformation measurements [32] . The lava discharge mechanism is thus responsible for the gas exsolution in deeper portions of the conduit, promoting the gradual upward rise in the gas-rich magma column [20] , [23] . This process is considered to be the cause of the decompression of the deep (7–10 km) [21] , [33] , [34] magma reservoir, which in turn triggered the rapid, buoyant rise of the crystal-poor, volatile-rich batch of magma during the 15 March violent ‘paroxysmal’ explosion [20] , [23] . However, we show that the volume of lava discharged during the effusive eruption follows the deepening of the VLP seismicity source ( Fig. 3 ), indicating that the magma supply rate from depth ( Q D ) was not sufficient to sustain the magma column level ( Q D < Q U ) within the conduit. This caused the continuous drainage of magma from the shallow reservoir and the lowering of the magma column during the effusive eruption. Thus, our model indicates that the magmastatic control of the shallow reservoir exerted an active role on the deep magma dynamics during the effusive phase. This also suggests that the inferred rise of the less dense and highly vesicular magma within the magma column [20] can be considered a possible consequence of the magma drainage from the shallow reservoir. The links between the position of the VLP seismicity, ground deformation and effusion rate allow us to quantify the magmastatic decompression, which ranges between 4.3 and 6.7 MPa. This offers a unique opportunity to derive the magnitude of the decompression rate from the ground tilt, which heavily influences our ability to predict the evolution of effusive eruptions at Stromboli. The magma drainage model by gravity load appears to dominate the effusive dynamics and changes our perspective from deep to shallow magma dynamics as the controlling factor for effusive eruptions. How to cite this article: Ripepe, M. et al . Volcano seismicity and ground deformation unveil the gravity-driven magma discharge dynamics of a volcanic eruption. Nat. Commun. 6:6998 doi: 10.1038/ncomms7998 (2015).